Electrografting of calix[4]arenediazonium salts to form versatile robust platforms for spatially controlled surface functionalization An essential issue in the development of materials presenting an accurately functionalized surface is to achieve control of layer structuring. Whereas the very popular method based on the spontaneous adsorption of alkanethiols on metal faces stability problems, the reductive electrografting of aryldiazonium salts yielding stable interface, struggles with the control of the formation and organization of monolayers. Here we report a general strategy for patterning surfaces using aryldiazonium surface chemistry. Calix[4]tetra-diazonium cations generated in situ from the corresponding tetra-anilines were electrografted on gold and carbon substrates. The well-preorganized macrocyclic structure of the calix[4]arene molecules allows the formation of densely packed monolayers. Through adequate decoration of the small rim of the calixarenes, functional molecules can then be introduced on the immobilized calixarene subunits, paving the way for an accurate spatial control of the chemical composition of a surface at molecular level. Surface functionalization has attracted considerable interest in recent years, with the aim to design surfaces with tailored properties (such as wettability, corrosion resistance, adhesion, lubricant, biocompatibility) or with operating functions ('smart' surfaces bearing stimuli-responsive architectures) [1] , [2] , [3] , [4] . When developed for modifying electrode surfaces, it finds applications in molecular electronics, [5] bioelectronics [6] , [7] , and in the development of charge transport devices [8] , [9] or sensors [10] . Particularly crucial for sensor studies, the controlled grafting of monolayers allows the design of complex recognition interfaces and provides responses akin to molecular level over the associated transduction reactions [11] . Three major issues for constructing such interfaces can thus be pointed out: control of the thickness and density of the deposited layer, which ideally, as a first step, requires the formation of a monolayer; spatial control of the connected functions and robustness versus temperature, solvents, ageing. The most popular strategy for fabricating monolayers is the spontaneous two-dimensional adsorption of thiol derivatives, especially alkanethiols, onto coinage metal (Pt, Au, Ag, Cu) forming self-assembled monolayers (SAMs) ( Fig. 1a ) [12] . Although highly versatile, this strategy could present important limitations related to their lack of thermal and long-term stability, narrow electrochemical window and stochastic behaviour of the gold–thiolate bond [12] , [13] , [14] . Besides, the spatial control of covalently bound functions is particularly difficult to achieve. Indeed, direct self-assembly of alkylthiols covalently connected at their extremity to functional objects generally leads to 'bouquet'-like repartition of the objects on the surface, with empty spaces in between ( Fig. 1b ) [12] . Dilution strategies with unfunctionalized alkylthiols allowing strong packing of the alkyl chain at the surface and simultaneous connection of large functional objects at the surface often lead to small 'islands of objects', not to regular distribution at the surface [12] , [15] , [16] , [17] , [18] , [19] . An alternative strategy for connecting organic moieties onto electrodes is the reductive grafting of aryldiazonium salts that yields covalent attachment of phenyl derivatives onto the surface. Electrografting in particular has gained tremendous interest over the last decade and is now a well-recognized method for surface functionalization [20] , [21] , [22] , [23] , [24] . Contrary to alkylthiol SAMs, the organic layers obtained from this method are generally highly stable, being strongly resistant to heat, chemical degradation and ultrasonication [20] , [25] . Furthermore, the method is easy to process and fast (deposition time on the order of 10 s instead of 10–18 h for well-organized thiol-Au SAMs) and can be applied to a wide range of materials: carbon (graphite, glassy carbon (GC), nanotubes, diamond), metals (Fe, Co, Ni, Cu, Zn, Pt, Au), semiconductor (SiH, SiO 2 , SiOC...), indium tin oxide and even organic polymers and dyes [22] . In spite of all these desirable properties, this strategy suffers from a major disadvantage, which is the poor control of layers thickness and regularity. Indeed, the reactive aryl radicals that are transiently produced attack not only the electrode surface but also already-grafted aryl layers, generally yielding multilayers and 'cauliflower'-like surfaces ( Fig. 1c ). This may result in the loss or decrease of efficiency of desirable properties, as observed for instance for the inferior charge transport properties of ferrocenyl redox moieties bound to such polyaryl layers [26] . 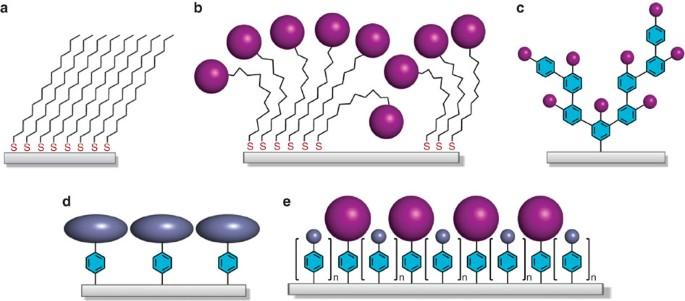Figure 1: Schematized strategies based on thiols and diazoniums for grafting organic layers onto surfaces. (a,b) SAMs (a) with simple alkylthiols, (b) bouquet-like layers with functionalized alkylthiols. (c–e) Diazonium methodology (c) cauliflower-like layers, (d) protection-deprotection strategy, (e) 'ideal' monolayers (see text for further explanation). Figure 1: Schematized strategies based on thiols and diazoniums for grafting organic layers onto surfaces. ( a,b ) SAMs ( a ) with simple alkylthiols, ( b ) bouquet-like layers with functionalized alkylthiols. ( c–e ) Diazonium methodology ( c ) cauliflower-like layers, ( d ) protection-deprotection strategy, ( e ) 'ideal' monolayers (see text for further explanation). Full size image Although the diazonium grafting could be empirically controlled to some extent through the appropriate choice of experimental conditions (nature of solvent, aryldiazonium salt concentration, electrolysis time and applied potential), an ultrathin and homogeneous coating is generally difficult to obtain, thus limiting the capability of the method in designing complex surface patterning. Introduction of sterically encumbered substituents on the aryl rings has been successfully used to prevent the uncontrolled polymerization process, thus allowing the formation of a near monolayer [27] . However, an undesirable counterback is the chemical inertness of these molecules, which precludes further functionalization. To remedy this problem, aryldiazonium salts bearing a pendant function masked by a protecting group exhibiting steric hinderance [28] , [29] , [30] , [31] and electronic shielding [29] properties have been used ( Fig. 1d ). After removal of the protecting group, a postfunctionalization step allows for the attachment of functional molecules onto the newly activated monolayer. However, because of the leftover void spaces between two adjacent grafted aryl molecules after the deprotection step, this two-step strategy could be disadvantageous when the direct formation of compact, pinhole-free layers is desired. A very recent article describes a more straightforward one-step strategy based on the reductive electrografting of a benzene( p -bisdiazonium) salt, leaving a pendant diazonium protecting group for further chemical coupling [32] . However, this route suffers from a lack of long-term stability of the diazonium-terminated layers. Here, we propose a different strategy based on surface pavement with versatile platforms that exhibit preorganization properties. This original concept uses rigid tetrapodant calix[4]arenes [33] as building blocks to form robust, closely packed and stable monolayers that can be postfunctionalized. Immobilization of calixarenes onto a surface by self-assembly techniques [34] is classically achieved by anchoring the small rim of the calixarenes onto the substrate through their phenol or thiophenol functions. In contrast, our strategy relies on the large rim grafting of calix[4]arenes, thanks to the diazonium coupling route, whereas the small rim is used for the introduction of spatially controlled postfunctionalizable groups. Adequate decorations of the small rim with appending arms make it possible to direct the introduction of functional molecules with a fine spatial control imposed by the geometry of the small rim, especially when two (or more) molecules are linked to the same calixarene. Close packing of the calix molecules and chemical control of the grafting process are ensured by the constrained cone conformation of the macrocycle that orients all four diazonium groups in the same direction and prevents polymerization of the transiently produced aryl radicals, thanks to the methylene bridges at the ortho-positions of the phenoxy substituents. It is noteworthy to mention that the preparation and the reductive grafting of calix[n]arenes fully substituted at the large rim by diazonium groups have never been reported. Synthesis and grafting procedures of calix[4]tetra-anilines p tBu-calix[4]arene was first O -alkylated by four alkyl or acyl groups following classical procedures. This allows to constrain the macrocycle in a cone conformation and to introduce at the small rim a carboxylic function that can easily be postfunctionalized. A sequence of ipso -nitration–reduction then yielded compounds 1 – 4 displayed in Fig. 2 (see the Supplementary Methods ) [35] . Non-postfunctionalizable calix[4]tetra-anilines 1 and 2 were first employed as model compounds for the surface modification and characterization, whereas compounds 3 and 4 were used to explore the postfunctionalization feasibility. 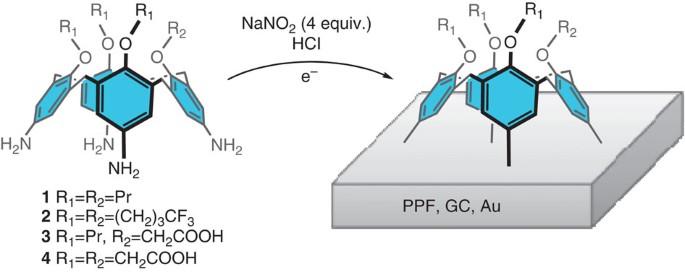Figure 2: Representation of the four calixarenes compounds undergoingin situtransformation to diazonium salts for electrografting. Structures of the calix[4]tetra-anilines (1–4) used in this work. The modification procedure of the gold, GC or PPF substrates relies on thein situdiazotation of the calix[4]tetraanilines in the presence of NaNO2in acidic aqueous medium followed by the electrochemical reduction of the corresponding diazonium salts. Figure 2: Representation of the four calixarenes compounds undergoing in situ transformation to diazonium salts for electrografting. Structures of the calix[4]tetra-anilines ( 1– 4 ) used in this work. The modification procedure of the gold, GC or PPF substrates relies on the in situ diazotation of the calix[4]tetraanilines in the presence of NaNO 2 in acidic aqueous medium followed by the electrochemical reduction of the corresponding diazonium salts. Full size image The grafting procedure was similarly conducted whatever the calix[4]tetra-aniline or the nature of substrate used. The corresponding diazonium salts 1 – 4 were prepared in situ in 0.5 M aqueous HCl in the presence of NaNO 2 (4 eq.) [36] . Gold, pyrolized photoresist film (PPF) or glassy carbon (GC) (disk electrodes) substrates were functionalized through the reduction of the in situ generated diazonium cations from calix[4]tetra-anilines 1 – 4 either by six voltammetric cycles or by applying a constant potential. 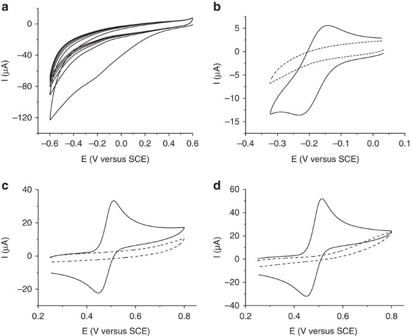Figure 3: Electrochemical answers at a GC electrode. (a) Cyclic voltammetry of calix[4]arene diazoniumin situgenerated from 5 mM calix[4]tetra-aniline 1 in 0.5 M aqueous HCl in the presence of 4 eq. NaNO2, scan rate 0.1 V s−1. The first cycle displays the reduction of diazonium cations; subsequent cycles (2–6) exhibit a clear decrease of the current. (b) Cyclic voltammetry of 1 mM Ru(NH3)63+/2+in 0.1 M KCl at a bare electrode (full line) and at a modified electrode after electrografting of2(dashed line). (c,d) Cyclic voltammetry of 1 mM Dopamine in 0.1 M H2SO4at a bare electrode (full line) (c,d) and at a modified electrode after electrografting of2(dashed line) (c) and after electrografting of4(dashed line) (d). Figure 3a shows a typical cyclic voltammogram for the electrografting of 1 on a GC electrode taken as an example. It exhibits the characteristic behaviour of the reductive electrografting of aryldiazonium salts [37] . The potential was swept between +0.6 V and −0.6 V versus saturated calomel electrode (SCE). On the initial potential cycle, a broad irreversible peak located at about −0.25 V versus SCE was observed then, a dramatic decrease of current intensity was recorded upon the following cycles. The peak stems from the reduction of diazonium cations into phenyl radicals that subsequently react at the electrode surface, forming a covalently linked blocking layer at the electrode interface. Alternatively, the reduction of the in situ generated diazonium cations was performed by applying a constant potential at –0.5 V versus SCE for 5 min. Figure 3: Electrochemical answers at a GC electrode. ( a ) Cyclic voltammetry of calix[4]arene diazonium in situ generated from 5 mM calix[4]tetra-aniline 1 in 0.5 M aqueous HCl in the presence of 4 eq. NaNO 2 , scan rate 0.1 V s −1 . The first cycle displays the reduction of diazonium cations; subsequent cycles (2–6) exhibit a clear decrease of the current. ( b ) Cyclic voltammetry of 1 mM Ru(NH 3 ) 6 3+/2+ in 0.1 M KCl at a bare electrode (full line) and at a modified electrode after electrografting of 2 (dashed line). ( c , d ) Cyclic voltammetry of 1 mM Dopamine in 0.1 M H 2 SO 4 at a bare electrode (full line) ( c , d ) and at a modified electrode after electrografting of 2 (dashed line) ( c ) and after electrografting of 4 (dashed line) ( d ). Full size image Characterization of the modified surfaces After copious rinsing with a series of solvents (water, ethanol, dichloromethane, toluene) and drying under a stream of argon, the grafted layers were characterized by analysing their blocking properties toward the electrochemical response of redox probes such as Fe(CN) 6 3−/4− ( Supplementary Fig. S1 ), Ru(NH 3 ) 6 3+/2+ and dopamine. Figure 3b–d shows typical voltammograms obtained with Ru(NH 3 ) 6 3+/2+ and dopamine from a GC electrode before and after electroreduction of the in situ generated diazonium cations from 2 or 4 . As compared with the reversible redox processes at the bare electrode, a complete inhibition of the electrochemical response of the grafted surface was evidenced for all the redox probes. This indicates that an organic layer was formed at the electrode surface, and that this layer acts as a barrier for redox processes. Particularly informative regarding the compactness of the layer is the behaviour of dopamine. Oxidation of dopamine to the corresponding o-quinone has been demonstrated to require adsorption onto the GC electrode surface for exhibiting fast charge transfer kinetics and it was established that the coverage of the electrode surface with a dense monolayer is enough to inhibit the oxidation of dopamine [38] . Thus, observation of an electrochemical activity implies that the molecular probe could reach the carbon substrate that makes dopamine oxidation a specific test for detecting pinholes [38] , [39] . In our case, we observed the complete inhibition of the dopamine redox activity after the grafting of calixarenes 2 and 4 layers. This observation demonstrates that the possible pinholes/defects/empty spaces within the grafted layers have size smaller than that of dopamine. To further characterize the grafted organic layer, contact angles of gold-modified substrates were measured using the sessile drop method ( Fig. 4 ). The static contact angle with water was found to be 78±3° for the surface modified with 1 and 89±2° for the surface modified with 2 , in comparison with the value of 62±2° for a bare gold surface. 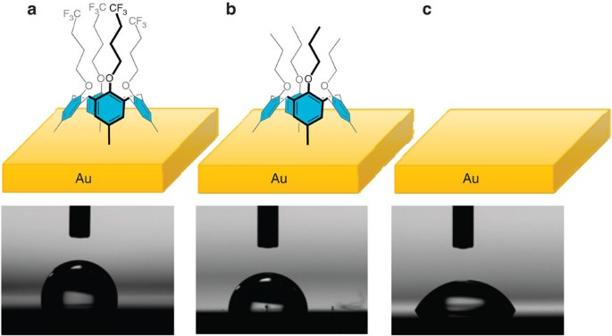Figure 4: Characterization of the modified gold substrates by contact angle measurements. Images of a 2 μl water droplet in contact with a gold substrate modified (a) with2, (b) with1and (c) on a bare substrate. Bare gold substrate is the most hydrophilic sample, showing that the droplet spreads out while the coated substrates, much less hydrophilic because of the grafted organic layer, show a different behaviour of the water droplet. Figure 4: Characterization of the modified gold substrates by contact angle measurements. Images of a 2 μl water droplet in contact with a gold substrate modified ( a ) with 2 , ( b ) with 1 and ( c ) on a bare substrate. Bare gold substrate is the most hydrophilic sample, showing that the droplet spreads out while the coated substrates, much less hydrophilic because of the grafted organic layer, show a different behaviour of the water droplet. Full size image These data indicate that hydrophobic films were formed on the gold surfaces due to the immobilization of the calixarenes. The larger contact angle for the surface modified with 2 is fully consistent with the stronger hydrophobic nature of the calix[4]arene 2 as compared with 1 . Remarkably, wetting studies for SAMs on gold formed with thio-calix[4]arenes yielded similar contact angle values [40] , [41] . X-ray photoelectron spectroscopy (XPS) analyses were performed on both PPF and gold substrates modified by the CF 3 -containing calix[4]tetra-aniline 2 , the CF 3 groups providing a convenient chemical tag for XPS studies. The survey spectra showed main peaks corresponding to the elemental species C, N and O, whereas peaks due to Au were observed on gold substrates ( Supplementary Fig. S2 ). In the case of gold substrates, an overall attenuation of the Au photoelectron peaks and a significant increase in the C1s and O1s peak heights, compared with the bare substrate, confirmed the coating of the gold substrate by an organic layer. A characteristic peak of the F1s photoelectrons appeared at 688.5 eV after surface functionalization by the calix[4]arene 2 . The presence of the CF 3 group was further confirmed by the emergence of a new component at 293 eV in the C1s core level spectrum ( Fig. 5 ). The C1s core level showed a main peak centred at 285 eV assigned to the aromatic carbons of the calix[4]arene phenyl groups (and to the carbon atoms of the substrate when analysing the PPF substrates). A component at 286.2 eV was also evidenced, which corresponds to the C–O environment present in the calixarene frame. The small components at the high binding energy side (at ~287.3 and 289 eV) accounts for oxidized carbon from contamination species already detected on the bare substrates. 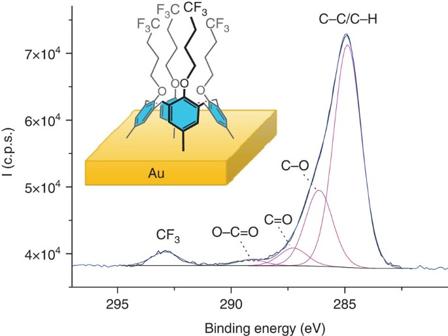Figure 5: High-resolution peak-fitted C1s region for gold substrate modified by calix[4]arene2. Surface composition is indicated in the integrated areas. Figure 5: High-resolution peak-fitted C1s region for gold substrate modified by calix[4]arene 2 . Surface composition is indicated in the integrated areas. Full size image The absence of a N1s peak attributed to –N 2 + (at 403.8 eV) indicates a complete transformation of the diazonium cations, whereas the very low intensity signal at 400 eV reveals the formation of a very small proportion of azo groups (–N=N–) derived from the diazonium salts as already reported in the literature [36] , [42] , [43] , [44] , [45] , [46] . Atomic force microscopy (AFM) analysis was performed by using preferentially PPF substrates because of their low surface roughness in comparison with GC or gold substrates employed in this work. PPF plates grafted with the reduction of diazonium cations issued from 1 or 2 showed surface structures almost identical and of same sizes as the bare PPF, indicating a uniform deposit on the whole surface ( Fig. 6 ). The surface roughness increased only slightly upon the electrografting of the calix[4]arenes (root-mean-square roughness, r.m.s.<1 nm) as compared with a bare PPF substrate (r.m.s.<0.8 nm) [47] . These observations fall in line with the formation of very thin layers. Remarkably, the surface roughness was not affected by electrolysis time (30 s, 1 min, 5 min, 10 min) employed for the electrografting of the in situ generated diazonium cations, suggesting that the system is self-inhibiting. 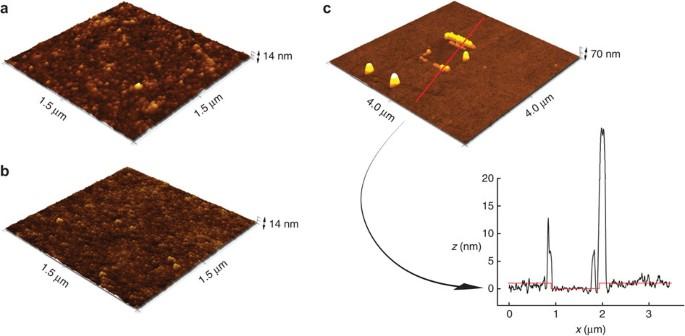Figure 6: AFM characterization of PPF sample modified with2. (a) AFM image (surface scale 1.5×1.5 μm2) of the bare PPF sample. (b) AFM image (surface scale 1.5×1.5 μm2) of the PPF sample afterin situgeneration and electrografting of diazonium cation from2. (c) Scratching of the PPF sample as imaged inb(surface scale 4×4 μm2). Depth-profile of the scratched area. Figure 6: AFM characterization of PPF sample modified with 2 . ( a ) AFM image (surface scale 1.5×1.5 μm 2 ) of the bare PPF sample. ( b ) AFM image (surface scale 1.5×1.5 μm 2 ) of the PPF sample after in situ generation and electrografting of diazonium cation from 2 . ( c ) Scratching of the PPF sample as imaged in b (surface scale 4×4 μm 2 ). Depth-profile of the scratched area. Full size image AFM technique was further used for estimating the thicknesses of the organic layers. The AFM tip was used in contact mode to scratch a rectangular area on the PPF functionalized samples by exercising a force sufficient to remove the organic part without damaging the PPF sample. Profiling depth measurements of the scratched area in an intermittent contact mode gave the average thickness of the layer, as described by Mc Creery and co-workers [48] . The thickness was thus estimated to be 1.3±0.1 nm ( Fig. 6c ). This result agrees well with the height of calix[4]arenes 1 and 2 ( c.a. 1.0 and 1.1 nm, respectively, estimated from MM2 energy minimizations with ChemBio3D software), and indicates that the electrografting of the corresponding diazonium cations led to the formation of monolayers. This result is further confirmed by ellipsometric measurements of gold substrates modified with calix[4]arene 2 . Thickness value of 1.09±0.20 nm was found, in very good agreement with the height of calix[4]arene 2 . Both techniques unambiguously demonstrate the formation of monolayers. From the strong blocking effect toward redox probe responses, namely regarding the answer of the monolayer towards dopamine, it can be further concluded that the formed monolayers are rather compact. Taking account the formation of monolayers, XPS data could be used to give a reliable estimation of surface coverage for the non-electroactive calixarene 2 . On gold samples, the average calix[4]arene coverage α on the gold surface could be expressed from F 1s and Au 4f peak intensities related to calix[4]arenes layers and the gold substrate, respectively [49] . The calculation (details provided in the Supplementary Methods ) leads to a surface coverage α of the gold substrate by the calix[4]arene 2 molecules of 79%. Calix[4]arenes present an external diameter of 14 Å (large rim) [50] . Considering a hexagonal compact arrangement of disks (or spheres) of 14 Å diameter, the surface concentration for the closest packing of calixarenes corresponds to Γ CPML =9.8×10 −11 mol cm −2 and the closest-packing monolayer covers 90.7% of the gold surface. It comes that the surface concentration of calixarene 2 onto gold substrate estimated from XPS data is equal to 8.5×10 −11 mol cm −2 (0.5 calix nm −2 ). All these results evidence the formation of a dense and compact monolayer of calixarenes. Postfunctionalization of the modified surfaces Having demonstrated the straightforward formation of monolayers from the electroreduction of diazonium cations derived from compounds 1 and 2 , calix[4]tetra-anilines 3 and 4 ( Fig. 7 ) were then used to modify substrates as a proof-of-concept for postfunctionalization purposes. The presence of one (for 3 ) or four (for 4 ) appending carboxyl group(s) at the calixarenes small rim allows a further chemical coupling using acyl chloride activation. Accordingly, ferrocene moieties were covalently introduced through an amide bond formation with ferrocenemethylamine (FcCH 2 NH 2 ) following a procedure previously described ( Fig. 7 ) [51] . 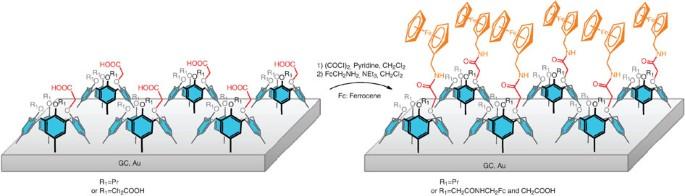Figure 7: Chemical postfunctionalization with ferrocenemethylamine of the calix[4]arene-modified substrates. The substrates were initially modified with calix[4]arenes3or4exhibiting one or four appending COOH groups at the small rim. The easy postfunctionalization is exemplified with the covalent binding of ferrocene redox centres. Figure 7: Chemical postfunctionalization with ferrocenemethylamine of the calix[4]arene-modified substrates. The substrates were initially modified with calix[4]arenes 3 or 4 exhibiting one or four appending COOH groups at the small rim. The easy postfunctionalization is exemplified with the covalent binding of ferrocene redox centres. Full size image After the chemical postfunctionalization, the modified substrates were thoroughly rinsed with CH 2 Cl 2 , then transferred to a pure CH 2 Cl 2 + 0.2 M NBu 4 PF 6 electrolyte solution. Well-defined oxidation and reduction peaks corresponding to the introduced ferrocene/ferrocenium couple were detected at c.a. 0.4 V versus SCE, as illustrated in Fig. 8 . It was also observed that the current linearly increased with scan rate in the (0.05–10 V s −1 ) range as expected for surface-confined electroactive species. 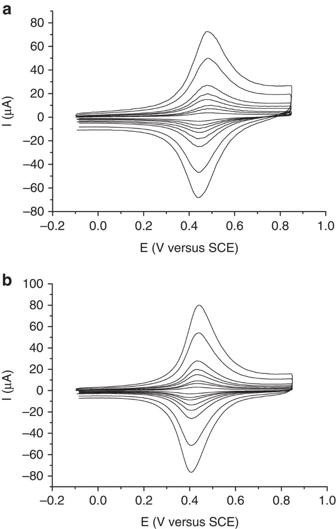Figure 8: Cyclic voltammetry of GC electrodes modified with calixarenes and postfunctionalized with ferrocene. The modified surfaces were obtained from the electrografting of diazonium cations of3(a) and4(b). CH2Cl2+0.2 M NBu4PF6. Ferrocene redox centres were covalently introduced on the calixarenes platforms from a chemical coupling using the COOH appending groups present at the small rim of calixarenes3and4. Cyclic voltammetry show the typical signal of surface-confined ferrocene centres. Scan rate varied from 0.1 to 3 V s−1. Figure 8: Cyclic voltammetry of GC electrodes modified with calixarenes and postfunctionalized with ferrocene. The modified surfaces were obtained from the electrografting of diazonium cations of 3 ( a ) and 4 ( b ). CH 2 Cl 2 +0.2 M NBu 4 PF 6 . Ferrocene redox centres were covalently introduced on the calixarenes platforms from a chemical coupling using the COOH appending groups present at the small rim of calixarenes 3 and 4 . Cyclic voltammetry show the typical signal of surface-confined ferrocene centres. Scan rate varied from 0.1 to 3 V s −1 . Full size image For experiments using calixarene 3 ( Fig. 8a ), the surface density of attached ferrocene centres was derived from integration of the voltammetric peaks at low scan rates. This allowed an estimation of the surface coverage of calixarenes themselves onto the substrate since each calixarene frame bears one functionalizable carboxyl substituent. Because the postfunctionalization reaction may not take place with 100% yield, this value could be regarded as a lower estimate of the calixarenes surface concentration. Surface concentration was found to be Γ 1 =6.9±0.6×10 −11 mol cm −2 , corresponding to a density of 0.42 calix nm −2 . This result is fully consistent with the surface concentration value estimated from XPS data and confirms the formation of rather densely packed monolayers, in line with the good blocking properties of the layers towards the electronic transfer. Note that the surface concentration here found is in good agreement with surface concentration reported for gold–thiols SAMs of calix[4]arenes [52] , [53] , or compares favourably with the density reported for the covalent and rigid grafting of calix[4]arenes onto silica surfaces [54] , the molecular footprint of the described calixarenes being similar to the calixarenes 1 – 4 . The surface concentration of electroactive ferrocene was similarly determined for experiments using the tetra-carboxylic acid decorated calix[4]tetra-aniline 4 . A surface concentration Γ 2 =1.6±0.4×10 −10 mol cm −2 was calculated. This surface concentration is one third the value reported for the closest packing of ferrocene [55] and corresponds to c.a. twice the Γ 1 value . This result indicates that two ferrocenyl moieties could be attached onto each calixarene subunit. This allows the introduction of functional groups on the surface with a precise spatial control, which is imposed by the calixarene small rim geometry. Calix[4]tetra-anilines have been successfully electrografted to various substrates by generating in situ their corresponding diazonium cations. Thanks to its well-preorganized and unique 3D conic structure, the calix[4]arene core prevents the formation of multilayers and leads to densely packed monolayers [56] . Characterization of the modified surfaces points out to an efficient packing of the calix molecules, probably ensured by the constrained cone conformation of the macrocycle that orients all four diazonium groups in the same direction. However, this does not necessarily imply that four aryl–substrate bonds are formed. This would depend on the availability of gold or carbon atoms sites and the possible degree of distortion of the calixarene molecule ( Supplementary Fig. S3 ). The important point is that the calix grafts with its cone axis perpendicular to the surface, whatever the number of aryl–substrate bonds formed, and the thicknesses reported in this work are in good agreement with this point. Providing that the calixarene platforms possess chemically reactive appending arms at the small rim, this strategy allows for the straightforward preparation of versatile robust monolayers that can be directed at the spatially controlled introduction of functional entities. This approach can be made even more sophisticated by using calix[4]arenes that exhibit two different anchoring termini on the same frame, thus opening new possibilities for the design of multicomponent films with a spatial control at the molecular level. Work is currently under way to implement this last approach. Synthesis The synthesis of the various calix[4]arenes compounds and their characterization are described in the Supplementary Methods . Surface modifications procedures The reagents and solvents used for surface chemistry were of high purity grade (Sigma-Aldrich, SDS, Alfa Aesar). The GC substrates were home-made disk electrodes of 3 mm diameter, thoroughly polished (successively with 5 μm SiC paper (Struers), 1 μm DP–Nap paper (Struers) with 0.3 μm Al 2 O 3 slurry (Struers)) and rinsed with ultrapure water, and absolute ethanol under sonication. Gold substrates (gold layer onto Si substrates) were purchased from Aldrich and thoroughly cleaned before surface functionalization (piranha solution). PPF samples were prepared according to previously published procedure [57] . Surface modification by electrochemical reduction of in situ generated diazonium cations was carried out in an ice bath. NaNO 2 (4 eq.) was added to the aqueous electrolytic solution containing 5 mmol −1 calix[4]tetra-aniline and 0.5 mol −1 HCl under stirring. After 5 min, the modification was achieved potentiostatically or by potential cycling between 0.6 and −0.6 V/SCE. After modification, the substrates were rinsed (sonication) with ultrapure water, abs EtOH, freshly distiled CH 2 Cl 2 and toluene (high-performance liquid chromatography grade). The subsequent ferrocenyl postfunctionalization was carried out according to ref. 51 . Electrochemistry Cyclic voltammograms were recorded with an Autolab electrochemical analyzer (PGSTAT 30 potentiostat/galvanostat from Eco Chemie B.V.) in a three-electrode setup with an SCE reference electrode and a platinum foil as counter electrode. The surface coverage of electroactive ferrocene is obtained from Faraday's Law, Γ= Q / nFA where Q is the charge passed, n the number of exchanged electrons, F the Faraday constant and A the area of electrode. Q is obtained from the integration of the area under the voltammetric peaks at low scan rates using the integration function of the Origin software. Polynomial baselines can be solved and subtracted before the curve integration. AFM microscopy analyses AFM experiments used a Picoscan II microscope (Agilent) coupled to a pico-SCAN2500 controller. The images were acquired in acoustic mode using silicon nitride tips (resonance frequency c.a 350 kHz). Scratching technique was used to determine the thickness of the organic layer grafted on the PPF samples. Square-shaped scratches were obtained in contact mode with a force set-point voltage around 1 V. Several depth-profiles were measured for each scratched region. Height distributions were also investigated on images to confirm the depth-profiles measurements. XPS measurements XPS photoelectron spectra were collected from modified GC and gold plates on a Thermo VG Scientific Escalab 250 system fitted with a monochromatic Al Kα X-ray source (hν=1486.6 eV, spot size=650 μm, power 15 kV×200 W). The pass energy was set at 150 and 40 eV for the survey and the narrow regions, respectively. Spectral calibration was determined by setting the main C1s component at 285 eV. The surface composition was estimated using the integrated peak areas and the corresponding Scofield sensitivity factors corrected for the analyzer transmission function. Contact angle measurements The static contact angles of 2 μl ultrapure water drops were measured on four different spots on the surface with an easy drop goniometer (Krüss). The contact angles were determined using a tangent 2 or circle fitting models. Ellipsometry Thicknesses of the layers on Au were measured with a mono wavelength ellipsometer Sentech SE400. The following values were taken for gold: n s =0.203, k s =3.431. These values were measured on clean surfaces before grafting and the layers thicknesses were determined from the same plates after modification, taking n s =1.5, k s =0 for the layer. Measurements reported are the average of ten data points across each substrate (two substrates were analysed). How to cite this article: Mattiuzzi, A. et al . Electrografting of calix[4]arenediazonium salts to form versatile robust platforms for spatially controlled surface functionalization. Nat. Commun. 3:1130 doi: 10.1038/ncomms2121(2012).